Superconductivity and its mechanism in anab initiomodel for electron-doped LaFeAsO Two families of high-temperature superconductors whose critical temperatures are higher than 50 K are known. One are the copper oxides and the other are the iron-based superconductors. Comparisons of mechanisms between these two in terms of common ground as well as distinctions will greatly help in searching for higher T c superconductors. However, studies on mechanisms for the iron family based on first principles calculations are few. Here we first show that superconductivity emerges in the state-of-the-art numerical calculations for an ab initio multi-orbital model of an electron-doped iron-based superconductor LaFeAsO, in accordance with experimental observations. Then the mechanism of the superconductivity is identified as enhanced uniform density fluctuations by one-to-one correspondence with the instability towards inhomogeneity driven by first-order antiferromagnetic and nematic transitions. Despite many differences, certain common features with the copper oxides are also discovered in terms of the underlying orbital-selective Mottness found in the iron family. Discovery of the iron-based superconductors in 2008 opened a new way to reach high-temperature superconductors [1] . It was found that there exist many similarities with other high- T c superconductors, namely the copper oxides; superconductivity occurs in iron (copper) layers upon carrier doping to the antiferromagnetic (AF) phase. (In a typical iron-based superconductor LaFeAs(O,F), the AF order is destroyed at the electron doping concentration δ =0.05, above which the superconductivity takes over.) However, significant dissimilarities also exist; one of significance is the active orbital degrees of freedom; five Fe d orbitals are involved near the Fermi surface in the iron-based superconductors, whereas in the copper oxides, only one Cu d orbital mainly constitutes the Fermi surface. Thus, one central issue of iron-based superconductors is the role of orbital degrees of freedom. Because of the nearby AF phase, many theoretical and experimental studies proposed that spin fluctuations play an essential role in stabilizing the superconductivity in common with proposals in copper oxides [2] , [3] , [4] , [5] , [6] , [7] . In particular, Platt et al. [7] discussed roles of magnetic fluctuations based on the first principles study combined with the functional renormalization group. Meanwhile, roles of orbital or nematic fluctuations were also suggested [8] , [9] . Although the normal state properties including magnetism were numerically analysed successfully in the iron-based superconductors [10] , [11] , the superconductivity has not been studied by quantitative ab initio calculations. Despite a large amount of research [12] , [13] , [14] , [15] , the primary cause that controls the high- T c superconductivity is still unresolved. Identification of the mechanism requires treating the spin and orbital degrees of freedom on an equal footing together with precise temporal and spatial quantum fluctuations. In the present study, we numerically study the ab initio low-energy effective models for the iron-based superconductors, particularly for electron-doped LaFeAsO by unprecedentedly large-scale computations, from which we identify superconducting mechanism in LaFeAsO. Our first interest is the significance of electron correlations [16] , [17] , [18] , [19] , [20] . In particular, the issue is whether the present ab initio study reproduces the proximity of the orbital-selective Mott insulator [21] , [22] , [23] , [24] , [25] , [26] , [27] , [28] , [29] , [30] , as was pointed out in the literature for the iron-based superconductors both from theoretical and experimental analyses [10] , [11] , [31] , [32] , [33] , [34] , [35] , [36] , [37] , [38] , [39] , [40] . A simpler perspective from a two-orbital model also exists [41] , [42] , [43] , [44] . It was established that a specific orbital , pinned close to half filling upon electron doping near the mother compound, LaFeAsO, shows a proximity to an orbital-selective Mott insulator [11] . This nearly Mott-localized orbital develops the AF order, where it couples to other orbitals by the Hund’s rule coupling and forms the high-spin moment. The origin of the orbital-selective Mottness on the ab initio grounds was interpreted from the higher density of states of the orbital at the Fermi level in the original bare band structure [11] . The higher density of states makes the orbital more sensitive to the interaction effect. We particularly focus on this orbital-selective behaviour as an underlying electronic structure that induces the superconductivity. Then the next important issue we examine is whether the superconductivity and its symmetry are correctly reproduced in the ab initio models for electron-doped LaFeAsO. The final and central issue is the mechanism of the superconductivity. Here we demonstrate first that the orbital-selective Mott insulating behaviour indeed emerges in our ab initio calculations for undoped LaFeAsO. Then we show that the electron doping eventually causes the depinning from the nearly Mott insulating orbital into metals triggering first-order AF transitions between high- and low-spin states. Filling-controlled first-order transitions generically drive inhomogeneity and phase separation. We next find that the superconductivity emerges in essential agreement with the experiments [1] , [6] . The pairing has a full gap and satisfies the symmetry with the opposite sign between the Fermi pockets at the Γ and M points in the Brillouin zone (so called s ± symmetry) [2] , [3] . Finally, we show by controlling the model parameters that the region of the strong density fluctuation near the phase separation remarkably has one-to-one correspondence with the identified superconducting regions. This smoking-gun observations support that the superconductivity in the iron-based superconductors is induced by the uniform charge (or in other words electron density) fluctuations discussed in the literature. The density fluctuation from the stripe-type AF order necessarily involves attraction of opposite spins at the next-neighbour bonds, which also generates the s ± singlet pairing. Thereby, generated superconductivity is stabilized by increased coherence of the carriers. Common and distinct features offer insights into the copper oxides as well. Model derivation and framework In showing the smoking gun of the superconductivity, we are based on an ab initio two-dimensional electronic model for LaFeAsO derived by using the downfolding procedure, which is detailed in the literature [45] . The ab initio Hamiltonian has the kinetic part and the interaction part as Here creates (annihilates) an electron with spin σ on the ν th Wannier orbital at the i th site. t i , j , ν , μ contains single-particle levels and transfer integrals. Details of and including transfer integrals and interaction parameters such as on-site intra-orbital/inter-orbital Coulomb interactions and exchange interactions are found in Methods, Supplementary Tables 1 and 2 , and in the literature [11] , [45] , [46] . The present model contains five Fe 3 d orbitals such as d XY , d YZ , , d ZX and . We note that the ( X , Y ) axis are rotated by 45° from ( x , y ) directed to the Fe–Fe direction. (for example, the direction of the d XY orbital is parallel to the nearest Fe–Fe direction.) To analyse the ground state of the ab initio model, we employ the many-variable variational Monte Carlo (mVMC) method [47] (see also Methods for details), which appropriately takes into account the strong correlation effects after considering both the quantum and spatial fluctuations. All the calculated extensive physical quantities are shown as those per site and the unit of the energy is eV, whereas the length unit is the nearest Fe–Fe distance. Detailed definitions of magnetic and superconducting quantities studied in the present work are given in Methods. Fully ab initio electronic model Now, we show results obtained by solving the fully ab initio electronic model. 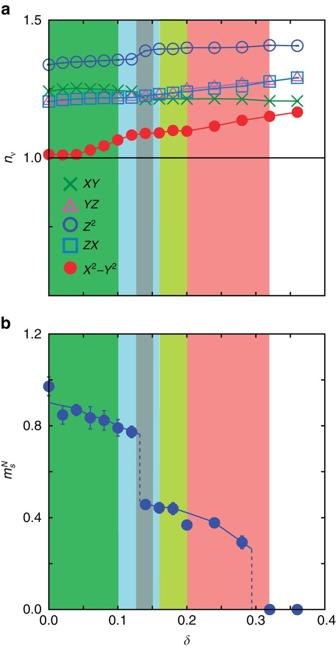Figure 1:  Orbital occupancies and AF order parameter ofab initioelectronic model. For definitions of coloured areas (phase diagram) and physical quantities, see alsoFig. 2and Methods. (a) Orbital-resolved filling as functions of doping concentrationδ. (b)δdependence of stripe-type AF order parameter for the normal state(filled blue circles), which indicates the AF order with large(LAF; dark green) and small(SAF; light green) phases. In all the figures hereafter, the error bars indicate the statistical errors of the Monte Carlo sampling. Curves are guides for the eye. Figure 1a shows the doping concentration ( δ ) dependence of the occupation of each orbital n ν for the normal state. Here δ =0 corresponds to the undoped mother compound LaFeAsO, where six 3 d electrons occupy an iron site on average. It clearly shows that the orbital (red filled circle) is pinned close to half filling upon electron doping from δ =0 to ~0.05 and the doping is small until the first-order transition at δ =0.13, indicating that the orbital stays nearly at the orbital-selective Mott insulator. The orbital selectivity in iron-based superconductors was discussed in several theoretical works [10] , [11] , [31] , [32] , [34] , [35] , [36] , [37] , [39] , [41] , [42] , [43] , [44] . We also find that the has the smallest double occupancy (see Supplementary Fig. 1a ), which indicates that the is located near the orbital-selective Mott insulator. The mechanism of the orbital differentiation in the ab initio model was discussed in ref. 11 as we mentioned above. The proximity of the orbital-selective Mott insulator is indeed confirmed in the present ab initio model at δ =0 as , , , , , where χ cν ≡d n ν /d μ is the orbital-dependent charge compressibility. The compressibility χ cν is prominently small for ν = X 2 − Y 2 as is expected from the proximity of the orbital-selective Mott insulator. Accordingly, near δ =0, it develops the stripe-type AF order as we see in Fig. 1b , where the largest contribution to the ordered moment comes from the orbital (see Supplementary Fig. 1b ) as is naturally expected as the Mott insulating nature of this orbital. Other orbitals are dragged by the orbital to the ordered state realizing the high-spin state, thanks to the Hund’s rule coupling J H (We confirmed that the AF order disappears even at δ =0 if orbital-dependent J Hνμ is uniformly reduced to 85% of the ab initio value.). Figure 1:  Orbital occupancies and AF order parameter of ab initio electronic model. For definitions of coloured areas (phase diagram) and physical quantities, see also Fig. 2 and Methods. ( a ) Orbital-resolved filling as functions of doping concentration δ . ( b ) δ dependence of stripe-type AF order parameter for the normal state (filled blue circles), which indicates the AF order with large (LAF; dark green) and small (SAF; light green) phases. In all the figures hereafter, the error bars indicate the statistical errors of the Monte Carlo sampling. Curves are guides for the eye. Full size image The electron doping destroys the AF order similar to the copper oxides. However, the suppression is initially slow because of the high-spin state, where the orbital blocking [10] does not seem to allow a gradual evolution of the kinetic energy gain. However, with the electron doping, this suppression of the kinetic energy gain is released by the transition to the lower-spin state, when the kinetic energy gain exceeds the energy gain by the Hund’s rule coupling. It easily occurs as a first-order transition as in other high-spin to low-spin transitions. This mechanism can be tested by directly calculating the off-site Green functions, which reflect the kinetic energy. The kinetic energy gain indeed suddenly increases at the first-order transition. As an example, we show the doping dependence of the nearest-neighbour orbital-diagonal Green functions in Supplementary Fig. 2 . We find that X 2 − Y 2 component of the Green’s function drastically increases around the first-order phase transition, which is consistent with above mechanism. Indeed, the high- to low-spin transition drives two successive first-order phase transitions; the first one occurs around δ =0.13 from large- m s AF (LAF) phase to small- m s AF (SAF) phase. The second one occurs around δ =0.3 between SAF and paramagnetic (PM) phases. As the stable phase, the second first-order transition is preempted by the emergence of the superconducting phase as we discuss later. We also confirmed that the nematic order that breaks the fourfold rotational symmetry to the twofold one coexists in the AF phase and shows a strong first-order transition simultaneously with the AF transition. After the first-order phase transition, we find that the nematic order seems to remain finite even in the PM phase. This may correspond to the electronic nematic phase observed in BaFe 2 (As 1− x P x ) 2 and Ba(Fe 1− x Co x ) 2 As 2 (refs 48 , 49 ), although it is not clear in LaFeAs(O,F) for the moment. In addition to the normal state, we now examine superconductivity: we started from various Bardeen–Cooper–Schrieffer-type superconducting wavefunctions that have different symmetries as the initial condition, and then relax and optimize all the variational parameters to lower the energy. After the optimization, we find that only the superconducting state with the gapped s ± -wave symmetry, which we call 3 s hereafter, survives. For detailed definitions of the superconducting states with 3 s symmetries and others, see Methods. In Fig. 2a , we show, by (red) triangles, the pairing order parameter of the gapped s ± -wave symmetry contributed from the orbital determined from the long-ranged (leveled-off) part of the pairing correlations, if it saturates to a non-zero value. Because the orbital gives the dominant contribution to ‹Δ 3 s › and contributions from other orbitals are small, we only show . The possibility of orbital-selective superconductivity has been discussed in the literature [50] . 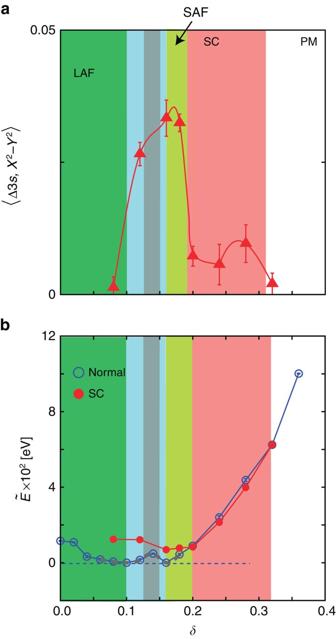Figure 2: Doping dependence of superconducting order parameter and total energies. (a)s-wave (gappeds±) superconducting order parameter of theorbitalin the superconducting phase. It is conspicuous thathas peaks around the first-order jumps of. SC indicates the superconducting phase. (b)δdependence of total energyof normal (blue circles) and superconducting (red circles) states. The ground state is superconducting for 0.2<δ<0.32 (red area). We subtracted a common linear termf(δ)=a+bδ(aandbare constants) from the bare total energy per siteE/Nsfor clarity. The spinodal region (see Methods) estimated as 0.12≤δ≤0.15 (grey region) is obtained by fitting aroundδ=0.13 up to the fourth polynomial (the bold grey broken curve). The phase separation region (0.1<δ<0.16 shown as light-blue area) is determined by the Maxwell’s construction (blue dashed line). The notations are the same asFig. 1. Figure 2: Doping dependence of superconducting order parameter and total energies. ( a ) s -wave (gapped s ± ) superconducting order parameter of the orbital in the superconducting phase. It is conspicuous that has peaks around the first-order jumps of . SC indicates the superconducting phase. ( b ) δ dependence of total energy of normal (blue circles) and superconducting (red circles) states. The ground state is superconducting for 0.2< δ <0.32 (red area). We subtracted a common linear term f ( δ )= a + bδ ( a and b are constants) from the bare total energy per site E / N s for clarity. The spinodal region (see Methods) estimated as 0.12≤ δ ≤0.15 (grey region) is obtained by fitting around δ =0.13 up to the fourth polynomial (the bold grey broken curve). The phase separation region (0.1< δ <0.16 shown as light-blue area) is determined by the Maxwell’s construction (blue dashed line). The notations are the same as Fig. 1 . Full size image This result indicates that the orbital governs the superconductivity as well as magnetism. In the sense that the single orbital plays a dominant role in stabilizing the superconductivity, it is similar to that of the copper oxides. The proximity to the half filling and its departure process of electrons in the orbital is a key to stabilize the superconducting phase. However, Fig. 2a also shows a crucial difference from the copper oxides. The superconducting order parameter shows dome structures near the strong first-order transition between LAF and SAF (as well as SAF and PM), where neither the AF nor the orbital (nematic) fluctuations show enhancement. At the first-order transition, the AF and nematic order parameters show a simple jump between the two rather doping independent values, which clearly show that their fluctuations are small. Therefore, the present ab initio result is difficult to reconcile with the spin/orbital fluctuation mechanism as the glue of the pairing. We will further inspect this correspondence between the first-order transition and the dome peak later. In Fig. 2b , we show δ dependence of the total energies E n and E s for the normal (open blue circles) and superconducting (filled red circles) phases, respectively. (Both are at least at local minima of the free energy for 0.08≤ δ ≤0.32.) For 0.2< δ <0.32 (red region), the superconducting state becomes the true ground state because E s < E n . From δ dependence of the total energy, the Maxwell’s construction, given by the broken thin blue straight line, determines the region of the phase separation 0.1< δ <0.16, where the thermodynamically stable and uniform phase is prohibited. Around the first-order transition at δ =0.13, the phase separation necessarily occurs when the filling is controlled because the phase coexistence occurs at the same chemical potential. The phase separation depicted by light blue and grey areas is an inevitable consequence of the first-order transition. Instabilities towards the phase separation are indeed experimentally observed in LaFeAsO 1− x F x (ref. 51 ) and Ba 1− x K x Fe 2 As 2 (refs 52 , 53 ), but in smaller regions. In addition, K x Fe 2− y Se 2 (ref. 54 ) and Rb x Fe 2− y Se 2 (ref. 55 ) suggest phase separation into iron-vacancy-ordered and iron-vacancy-free regions, possibly driven by the underlying electronic phase separation into AF and superconducting regions. In terms of the present result, it is intriguing to examine in more detail the uniformity of the other iron-based superconductors that do not show clear evidences for the phase separation so far. A small spinodal region (grey region) is seen, where the second derivative of energy with respect to density is negative meaning the thermodynamically unstable region (see Methods). In the region between the phase separation (light blue) and the superconducting (red) regions, we find a stable SAF (light green) region that has a small moment . The emergence of the superconducting dome upon electron doping after the destruction of the stripe-type AF order qualitatively and essentially reproduces the experimental phase diagram [1] , [6] . Therefore, it is now desired to clarify the origin of this superconductivity. Before discussing the superconducting mechanism, however, it should be noted that the obtained phase diagram looks quantitatively different from the experimental phase diagram of LaFeAs(O,F) in which AF and phase separation are limited to smaller doping regions. We discuss the origin of these discrepancies below. Effects of controlling electron correlations To understand correlation effects on the phase diagram in more general, we monitor the interaction by introducing the uniform scaling parameter λ only for the interaction part as Namely, λ =1 represents the original ab initio electronic model. For λ =0.95, as a function of δ , the magnetic ordered moment m s and superconducting order parameter are plotted in Fig. 3a and the total energy is shown in Fig. 3b . The dome of again appears near the first-order transition. However, it turns out that a small change of λ induces a drastic change, where the AF region largely shrinks to 0< δ <0.04 and the phase separation region in the normal state is replaced with the stable superconducting phase in the region 0.04< δ <0.08. 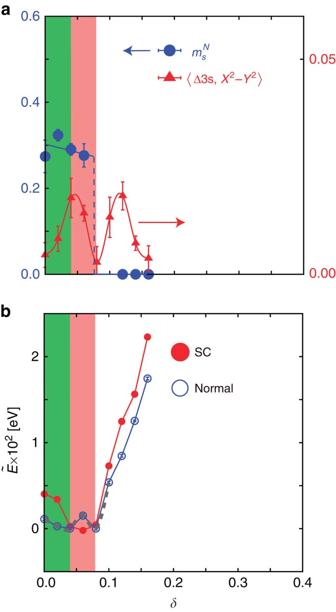Figure 3: Doping dependence of AF order parameter, superconducting order parameter and total energies atλ=0.95. (a) Doping concentration dependence of stripe AF orderin the normal state (blue circles) and the superconducting order parameter in the superconducting state (red triangles). (b) Total energies per site for normal and superconducting phases as functions ofδ. The notations are the same asFigs 1and2. Figure 3: Doping dependence of AF order parameter, superconducting order parameter and total energies at λ =0.95. ( a ) Doping concentration dependence of stripe AF order in the normal state (blue circles) and the superconducting order parameter in the superconducting state (red triangles). ( b ) Total energies per site for normal and superconducting phases as functions of δ . The notations are the same as Figs 1 and 2 . Full size image In Fig. 4 , we draw the global phase diagram in the λ – δ plane obtained by extensive calculations. It is noteworthy that the experimental phase diagram of LaFeAs(O,F) is consistent with that at a parameter λ between 0.95 and 1.0 in terms of the regions of the magnetic stripe order with the moment and the superconducting dome. The strong first-order transition between the stripe AF and superconducting phases at δ =0.05 is also consistent with the experimental phase diagram. In LaFeAs(O,F), the phase diagram shows an orthorhombic-tetragonal structural transition nearly at the magnetic-superconducting transition. As the electron-lattice coupling is not considered in the present ab initio model, the structural transition cannot be reproduced. Nevertheless, the present result supports that the orthorhombic-tetragonal transition is driven by the transition of the nematic order accompanied by the magnetic transition, which supports that the first-order transition is driven by the electronic mechanism. 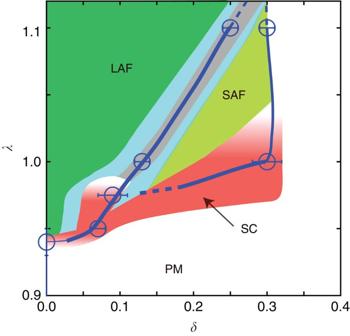Figure 4: Phase diagram inλ−δplane. Hereλis the parameter to scale the interaction energy andδis the doping concentration. Atδ=0, AF order parameter continuously vanishes atλ=0.94. Red region represents the superconducting phase, whereas the LAF and SAF phases are drawn as dark and light green areas, respectively. Grey area represents the spinodal region sandwiched by the light-blue phase separation region. Blue curves represent the magnetic transition lines in the normal phase, which are preempted when it is located in the spinodal (grey) or superconducting (red) regions. The transition is mostly of first order (bold curve) except for the region very close toδ=0, where it looks continuous. Figure 4: Phase diagram in λ − δ plane. Here λ is the parameter to scale the interaction energy and δ is the doping concentration. At δ =0, AF order parameter continuously vanishes at λ =0.94. Red region represents the superconducting phase, whereas the LAF and SAF phases are drawn as dark and light green areas, respectively. Grey area represents the spinodal region sandwiched by the light-blue phase separation region. Blue curves represent the magnetic transition lines in the normal phase, which are preempted when it is located in the spinodal (grey) or superconducting (red) regions. The transition is mostly of first order (bold curve) except for the region very close to δ =0, where it looks continuous. Full size image The consistency with the experimental result at λ ~0.97 implies a slight (<5%~0.1 eV) overestimate in the ab initio values of the interaction, which could arise from the possible error in the downfolding procedure, and we conclude the essential agreement between the calculated result with the experiment. Furthermore, beyond the present electronic ab initio scheme, such a small reduction of the effective interaction may arise from the electron–phonon interaction, where the frequency-dependent effective attraction was estimated as 0.4 eV but only within the range of the Debye frequency ~0.02 eV (ref. 56 ). The AF phase disappears and the superconductivity emerges in the mother compound LaFePO (ref. 57 ). This is again consistent with the present phase diagram as the ab initio model of LaFePO corresponds to λ <1 and δ =0 (ref. 11 ). By increasing λ beyond 1.0, the AF phase becomes quickly wider up to δ =0.3. This sensitivity to the interaction may account for recent experimental results of LaFeAsO 1− x H x , where the AF phase reappears in the overdoped region δ ≳ 0.4 (refs 58 , 59 ). Actually, it is reported that hydrogen substitution increases the anion height around δ =0.5 (ref. 60 ). The increase enhances the effective interactions because the screening from the anion p orbitals becomes poorer [45] . The reappearance of the AF phase in LaFeAsO 1− x H x accounted in this way is an interesting future subject of the first principles study. Control of off-site interactions To get further insight into the superconducting mechanism, let us study the ab initio model but here by switching off the off-site interactions V nn and V nnn . The ground states again contain the LAF (0< δ <0.1), SAF (0.15< δ <0.24) and superconducting phases (0.24< δ <0.32), as well as the spinodal (0.1≤ δ ≤0.15) region under the constraint of uniformity, which are not appreciably different from the ab initio model. However, the phase separation region is substantially widened to 0.08≤ δ ≤0.3 as we see in Fig. 5a . Therefore, all of the SAF phase and most of the superconducting phase (0.24< δ <0.3) become preempted by the phase separation region. Although the superconducting order parameter is substantially increased by switching off the off-site Coulomb interactions as we see in Fig. 5b , the stable superconducting region substantially shrinks and appears only near δ =0.32 because of the widened phase separation region. This result shows that the off-site Coulomb interactions are harmful for superconductivity in this case. 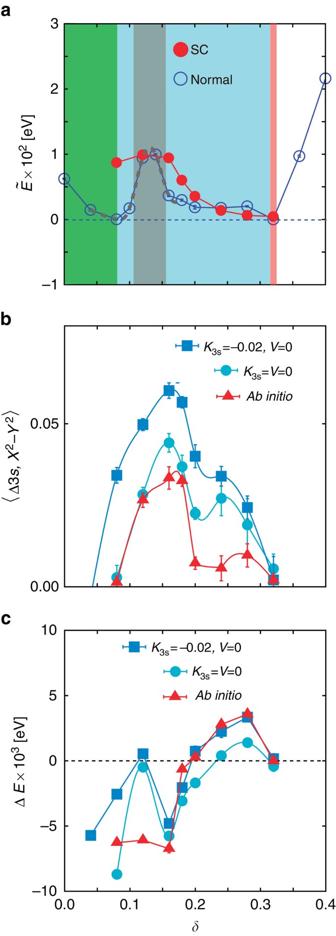Figure 5: Doping dependence of total energies, superconducting order parameters and condensation energies by controlling off-site interactions. The notations are the same asFigs 1and2. (a)δdependence of total energy for normal (En, open circles) and superconducting (Es, filled circles) phases forab initiomodel but by switching off off-site interactions. The Maxwell’s construction (blue broken line) determines the phase-separated region as 0.08≤δ≤0.32. (b) Comparison of superconducting order parameteramong theab initiomodel (triangles), the model without off-site interactions (circles) and a model with an added attractionK3s=−0.02 eV (squares). (c)δdependence of the energy difference between the superconducting and normal states (ΔE=En−Es) for the same cases as those inb. Figure 5: Doping dependence of total energies, superconducting order parameters and condensation energies by controlling off-site interactions. The notations are the same as Figs 1 and 2 . ( a ) δ dependence of total energy for normal ( E n , open circles) and superconducting ( E s , filled circles) phases for ab initio model but by switching off off-site interactions. The Maxwell’s construction (blue broken line) determines the phase-separated region as 0.08≤ δ ≤0.32. ( b ) Comparison of superconducting order parameter among the ab initio model (triangles), the model without off-site interactions (circles) and a model with an added attraction K 3 s =−0.02 eV (squares). ( c ) δ dependence of the energy difference between the superconducting and normal states (Δ E = E n − E s ) for the same cases as those in b . Full size image It was reported that the off-site interaction dramatically suppresses the superconductivity in the single-band Hubbard model [61] , whereas it is not in the present case. The origin is that the robust first-order magnetic transition stabilized by the Hund’s rule coupling cannot be suppressed by the off-site interaction here. This keeps wide area of enhanced charge fluctuations as we see later, although the phase separation itself is suppressed. We also add an explicit attraction, by replacing the off-site interactions to see more clearly how the pairing correlation is stabilized. Figure 5c shows that the superconductivity is stabilized in a wider region (0.2< δ <0.32) even at V nn = V nnn =0, when a small attraction K 3 s =−0.02 eV defined in Methods is added, which may represent an electron–phonon interaction phenomenologically but rather exaggeratingly. The enhanced superconducting order parameter is also seen more clearly in Fig. 5b in a wider region (0.04< δ <0.32). These rather artificial analyses are helpful in extracting the origin of the superconductivity as detailed below. The crucial roles of the onsite interaction and the Hund’s rule coupling in stabilizing the superconductivity are clear because the magnetic order itself is suppressed when they are weakened as clarified already [11] , which destroys the underlying playground of the first-order transition. On the other hand, as is evident in Fig. 5b , the off-site interaction suppresses the superconducting order. Smoking gun for superconducting mechanism Now by collecting all the results from different parameters that provide diverse phase diagrams, we show that the instability towards the phase separation unexceptionally enhances the superconducting order without ambiguity. In Fig. 6a , δ dependence of the superconducting order parameter is compared with the negative of the inverse charge compressibility −1/ κ defined from the second derivative of the energy with respect to δ , 1/ κ ≡ d 2 E s / dδ 2 for all the cases we studied including the fully ab initio model. These two quantities show a good and one-to-one correspondence, supporting the mechanism in which the charge fluctuation originally arising from the phase separation signalled by 1/ κ <0 and associated with the first-order magnetic/nematic transition is required for the emergence of the superconductivity of the iron-based superconductors LaFeAsO. This result is a direct evidence that the charge fluctuations induce the superconductivity. 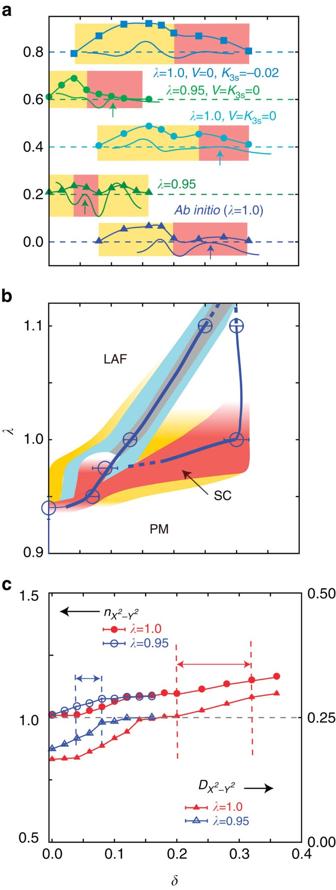Figure 6: Analysis on smoking gun for superconductivity. (a) Comparison ofδdependence of the superconducting order parameter(symbols) with(curves without symbols) for various models. The ordinates have 0.2 off-set (dashed line) in sequence for clarity. The yellow and red regions indicate non-zero. The peaks ofand−1/κshow one-to-one correspondences. Furthermore, the stable superconducting phase (red) emerges always when 1/κtends to vanish. (b) The region of non-zero(either stable (red) or metastable (yellow)) surrounds the first-order transition accompanied by the phase separation. (c) Comparison of stable superconducting phase (two-sided arrows) with the density, and the double occupation. Figure 6b further demonstrates that non-zero superconducting order emerges consistently around the region of the phase separation centred at first-order transition line. Figure 6: Analysis on smoking gun for superconductivity. ( a ) Comparison of δ dependence of the superconducting order parameter (symbols) with (curves without symbols) for various models. The ordinates have 0.2 off-set (dashed line) in sequence for clarity. The yellow and red regions indicate non-zero . The peaks of and−1/ κ show one-to-one correspondences. Furthermore, the stable superconducting phase (red) emerges always when 1/ κ tends to vanish. ( b ) The region of non-zero (either stable (red) or metastable (yellow)) surrounds the first-order transition accompanied by the phase separation. ( c ) Comparison of stable superconducting phase (two-sided arrows) with the density , and the double occupation . Full size image In Fig. 6c , the region of the stable superconducting phase (two-sided arrows) is compared with the orbital-resolved filling and the double occupation for two cases (the ab initio model ( λ =1) and the case at λ =0.95). The stable superconducting regions are found when and grow fast, indicating the importance of the transient region in the process to reach the quasiparticle coherence for the electrons in the X 2 − Y 2 orbital. Although the charge fluctuation enhances the superconducting order, not only the non-zero superconducting order parameter but also the coherence of the orbital carrier is required to truly stabilize the superconducting phase. This is the reason why the stable superconductivity asymmetrically appears at δ larger than that of the first-order transition, whereas at smaller λ ( λ =0.95), the coherence is already expected at small δ , where the superconducting region appears symmetrically around the magnetic transition. Here we discuss a possible mechanism of the superconductivity that is consistent with the present results indicating the one-to-one correspondence in Fig. 6 . Our result shows that the superconductivity emerges in the region where the strong first-order magnetic/nematic transition occurs, and the magnetic/nematic fluctuations are small. Thus, among several possible candidates of the pairing glue studied before and introduced in the beginning of this article, spin and orbital fluctuations are not supported. The only possible prominent fluctuations are the density fluctuations. When we switch off the off-site Coulomb interactions, we find that both the phase separation and the superconducting phase are enhanced while magnetic order changes little. This result also indicates the relevance of the density fluctuations. Indeed, the superconductivity from the phase-separation fluctuation was proposed by Emery, Kivelson and Lin as the mechanism of superconductivity in the copper oxides [62] . A general mechanism was discussed from the quantum critical fluctuation arising from the first-order transition of the density [63] . Recent numerical calculations for the Hubbard model also suggest the importance of the uniform charge fluctuations in stabilizing the superconductivity [61] . In this mechanism, the instability around the spinodal decomposition must necessarily cause the attractive effective interaction of the carriers, because the coefficient of the quadratic term with respect to the density has to be negative in the energy around the spinodal point. It is known that the attractive interaction of the carrier is the direct cause of the pairing (whatever the origin of the attractive interaction is) and is very natural to induce the superconductivity, if the carriers are in the Fermi degeneracy region. One can argue that the low-energy excitation associated with the translational symmetry gives density fluctuations, which may play the role of the glue even when they are not gapless. However, this is not so straightforward because the superconductivity competes with the phase separation or other density orders. Therefore, we need reliable quantitative calculations how the superconductivity wins or is defeated by considering quantum fluctuations as much as one can do. Our ab initio studies by the variational Monte Carlo calculation show that the superconductivity indeed wins in a relevant region. Our conclusion is that among possibilities, the result supports that the uniform charge fluctuations lead to the superconductivity observed in LaFeAs(O,F). For iron-based superconductors, a charge-fluctuation mechanism was also proposed in a different context in the model with Fe 3 d and pnictogen (chalcogen) p orbitals [64] . We note that the strong first-order transition by the carrier density control is of course not a sufficient condition for the realization of the superconductivity. Combination with the (orbital selective) Mottness is important, where the effective attractive interaction should take place between spin-1/2 carriers. This is a crucial difference from other first-order transitions accompanying phase separation such as those found in perovskite manganites with the double exchange mechanism. Here the uniform charge fluctuations signalled by the enhanced −1/ κ indicate the tendency for the aggregation of the antiferromagnetically coupled high-spin region segregated from the low-moment spins similar to the case of the liquid–gas (or binary alloy) transition. The aggregation must be mediated by the attraction of the high-moment up and down spins (or equivalently attraction of the low-moment spins) in the stripe-type configurations. In the stripe configuration, the two mutually 90° rotated configurations are degenerate and they interfere destructively for the nearest neighbour pair. However, the two stripe configurations are both constructively enhanced by the attraction of opposite spins at the next-nearest neighbour bonds. This attraction causes the s ± Cooper pair as well. Namely, the phase segregation and the singlet pairing with the s ± symmetry are two-sides of coins and are simultaneously driven by the next-neighbour attraction of the pair caused by the high- to low-spin transition and the underlying rapid Mottness crossover. The mechanism we revealed may be experimentally tested by measuring the superconductivity at the interface of two bulk superconductors with different doping concentrations, one being the mother material with AF order and the other being the overdoped non-superconducting materials as in the experiment for the interface of the cuprate superconductors [65] . When the average electron density of the interface is tuned around the phase separation region, we predict that the transition temperature is kept constant at the optimum value [61] . In fact, in the thin film of FeSe on SrTiO 3 , high- T c superconductivity ( T c ≳ 50 K) was reported [66] . The phase separation in A x Fe 2− y Se 2 , ( A =K, Rb) [38] , [40] , [54] , [55] into AF and superconducting regions with a high critical temperature above 60 K was also reported in experiments. These are also consistent with the present results, because the optimum doping concentration can be realized near the interface of the two phases. The systematic study on the electron concentration dependence at the interface will clarify more clearly the mechanism revealed here. We have not discussed the role of magnetic fluctuations in detail. This is because, around the strong first-order transitions, the magnetic fluctuations are not significant as we already discussed. Near the magnetic quantum critical point around λ =0.94 seen in Fig. 4 , however, the magnetic fluctuations are expected to contribute, whereas the density fluctuations are suppressed because of the conversion of the first-order transition to a continuous one. Indeed, the functional renormalization group study combined with the first-principles approach similar to ours suggests the role of magnetic fluctuations [7] . The functional renormalization group is a complementary weak-coupling approach, where weak instability to the superconductivity can be easily studied. The mVMC is able to study more easily the strong coupling superconductivity. We, however, see in Fig. 4 that the superconducting phase is extended even to the region around the quantum critical point, implying the applicability of mVMC in both strong and weak coupling regions. In most of the phase diagram, the density fluctuations play the dominant role in stabilizing high- T c superconductivity as the strong coupling mechanism. More quantitative ab initio analyses including other families of the iron-based superconductors and the role of phonons as well as guiding principle for raising T c are intriguing and challenging issues left for future studies. Details of model Hamiltonian In the present approach, we seek for an undoubted way of extracting the origin and mechanism of the experimentally observed superconductivity in the iron-based superconductors based on material-dependent realistic calculation. For this purpose, we employ the ab initio way of deriving the effective Hamiltonian without any adjustable parameters. Then, we solve the effective model as accurate as possible within the available methods. The Hamiltonian of low-energy effective model for a two-dimensional layer of LaFeAsO is given by Here t i , j , ν , μ contains single-particle levels and transfer integrals, whereas U i , i , ν , μ and J i , i , ν , μ are screened Coulomb and exchange interactions, respectively. The exchange interaction J i , i , ν , μ consists of the Hund’s rule coupling (conventionally denoted as J Hνμ ≡ J i , i , ν , μ ) in the first term and the pair hopping in the second term. We use the transfer integrals up to the fifth neighbours [45] , which well reproduce the local density approximation (LDA) band structures. In the off-site Coulomb interactions H off-site , V nn ( V nnn ) represents the nearest-neighbour (next-nearest-neighbour) Coulomb interactions and n iν denotes the orbital occupation of ν th orbital at the i th site [45] . From the ab initio downfolding procedure, we estimate V nn =0.4 eV and V nnn =0.2 eV (ref. 46 ). Further neighbour interactions are exponentially small because the two-dimensional effective model takes into account metallic screening from other layers. Because the off-site interactions do not appreciably depend on the combinations of orbitals and are distributed within 0.01 eV, we ignore the orbital dependence. Other off-site interactions such as the off-site direct exchange interactions are also less than 0.01 eV on average and we also ignore them. All of the model parameters were derived in the so-called downfolding procedure [45] . In this procedure, the global electronic structure is calculated by the ab initio density functional calculations. Then, the degrees of freedom whose energies are located far away from the Fermi level are traced out, leaving the ab initio effective model appropriate near the Fermi level, namely, for Fe 3 d five orbitals on the experimental crystal structure. Then, the ab initio two-dimensional model for a layer, where Fe atoms are arrayed on a square lattice, is derived after the dimensional downfolding [46] . The detailed description of the Hamiltonian parameters are found in refs 11 , 45 , 46 . The doping concentration ( δ ≡1− N e / N s ) dependence is studied in this article by changing the electron number N e in a layer containing N s iron sites in the periodic boundary condition, where other parameters in the Hamiltonian are assumed to be fixed through the doping process. Although it is adequate within the present work, in the main text, we also discuss possible modification of the Hamiltonian parameters by heavy doping. Details of mVMC We study the possibility of superconductivity in the model (5)–(9) by a mVMC method formulated in the literature [47] . In the mVMC calculations, we study the ground-state properties by employing a generalized Bardeen–Cooper–Schrieffer-type wave function with the quantum number projection and the Gutzwiller [67] and Jastrow factors [68] ; . Here, is the spin projection operator to the total spin S =0 subspace; and are the Gutzwiller and Jastrow factors, respectively [47] . The spin projection is performed onto the S =0 singlet subspace. The Gutzwiller factor punishes the double occupation of electrons by , where . The Jastrow factor is introduced up to the next-nearest-neighbour sites as , where n iν =σ σ n iνσ . The one-body part ∣ φ pair ∣ is the generalized pairing wave function defined as , where N e is the number of electrons. In this study, we restrict the variational parameters, g iν , v ijνμ to have a 2 × 1 structure, and f ijνμ to have a 2 × 2 sublattice structure. The number of variational parameters are 10 for g iν , 220 for v ijνμ and 100 N s for f ijνμ . All the variational parameters are simultaneously optimized by using the stochastic reconfiguration method [47] , [69] . Our variational wave function can flexibly describe superconducting, AF and PM phases as well as their fluctuations on an equal footing. The calculations were done up to 10 × 10 sites. Monte Carlo sampling of real space configurations of the electrons is employed to calculate physical quantities following the standard procedure [47] . The acceptance ratio of the Monte Carlo sampling is typically more than 10%. Here we define the autocorrelation as where n σ ( r i , t ) the number of particle at i th site, and t represents Monte Carlo step. is the averaged density per spin, which is defined as . The autocorrelation vanishes within 10–20 Monte Carlo steps. We show an example of A ( t ) in Supplementary Fig. 3 . The number of Monte Carlo samples for the calculation of physical quantities is typically 128,000. The statistical error of the Monte Carlo sampling is estimated from a number of independent bins typically around five. Details of physical properties To reveal physical properties and determine the phase diagram of the ab initio model, we calculated orbital-resolved filling n ν , orbital-dependent double occupation D ν , equal-time spin structure factors m ( q ) 2 , its orbital-diagonal component m ν ( q ) 2 , the equal-time superconducting correlation P α ( r ) and its orbital-resolved component P α , ν , μ ( r ), which are defined as where σ represents Pauli matrix. In actual calculations, to reduce numerical cost, we restrict the summation with respect to r i within 2 × 2 sublattice. The magnetic order parameter is estimated after the size extrapolation of the finite size data from 4 × 4 to 10 × 10 to the thermodynamic limit. The extrapolation is performed as a linear fitting of m ( Q ), as a function of the inverse linear dimension 1/ L , where Q is the peak position of m ( q ). Stripe order is determined from the Bragg peak at (0, π ), or (π, 0). Superconducting order parameter and its orbital diagonal component are defined as Here f α ( r ) is the form factor that describes the symmetry of the superconductivity. In the present work, we examined the four possible symmetries of the superconducting states; α =2 s (gapless s ± ), , 3 s (gapped s ± ), and 3 d ( d xy ), whose form factors are defined as where δ i , j denotes the Kronecker’s delta and r =( r x , r y ). We mainly study the case of f α with α =3 s often called s ± symmetry, where the pairing is between the electrons on the next-nearest-neighbour sites, because this symmetry of the pairing is the only one that survives in the realistic model. The nodal struture of this pairing is shown in Supplementary Fig. 4a . Initial conditions with other symmetries converge to the normal state. The order is determined from the long-ranged level-off part of the averaged pairing correlation , where we omit the contribution from the orbital off-diagonal pairing, because they are expected to be smaller. In Supplementary Fig. 4b , we plot the superconducting correlation P 3 s , ν ( r ) for an example of ν = X 2 − Y 2 as a function of the distance for the superconducting phase for the ab initio model at δ =0.24. In the normal phase, the superconducting correlation shows a power-law decay (~ r −3 ), and its amplitude is comparable to that of the non-interacting case. In contrast to this, in the superconducting phase, the superconducting correlation is saturated to a non-zero constant value as in Fig. 1b . To see whether the superconducting correlation is saturated to a non-zero value, we define long-range average of the superconducting correlation as where M is the number of vectors satisfying ( L is a linear dimension of the system size). For the present purpose, R =3 is practically a sufficient criterion to see whether the pairing order-parameter correlation is saturated to a non-zero value and offers a good measure for the order parameter in the long-range ordered superconducting state. To further reduce the finite size effect, we subtract calculated for the normal state from that for the superconducting state . In the actual calculations, in the normal state is non-zero because of the finite size effects. In the analyses, we use . We observed that is always dominant over other orbital contributions. Details of attractive interactions When we examine the effects of attractive interactions, we add an attractive interaction term, defined as where Δ 3 s , ν ( i ) represents the superconducting order parameter of ν th orbital at i th site for the gapped s ± -wave superconductivity. Similar interactions can be derived by considering the phonon degrees of freedom [70] . In actual calculations, we dropped the one-body part that originates from the commutation relation. We also dropped the AF interactions term that is proportional to S i · S j and contained in equation (19), which induces the AF order. Details of phase diagram The phases in the phase diagram are determined by the lowest energy state if more than one locally stable states are found. The stripe type magnetic order with the large (small) ordered moment is shown as dark (light) green area and the superconducting phase is shown as red area in the figures of the main text. In addition, thermodynamically prohibited region by the phase separation (phase separation region; illustrated as light blue areas in the figures) is determined by the Maxwell’s construction, where the region of the ground-state energies above a common tangent of the two points in the δ dependence of the ground-state energy is identified as the phase separation region. If the second derivative of the energy d 2 E / dδ 2 is negative inside the phase separation region, the region is locally unstable to inhomogeneity even under an infinitesimal perturbation and called spinodal region (grey area in the figures). The phase separation and accompanied spinodal region are natural consequences of the first-order magnetic transitions. Strictly speaking, the stable uniform states are prohibited in the spinodal region in the thermodynamic limit. Precise estimate of the spinodal region from the calculation of finite-size systems is difficult, because the negative curveture of the energy is eventually prohibited in the thermodynamic limit. How to cite this article : Misawa, T. and Imada, M. Superconductivity and its mechanism in an ab initio model for electron-doped LaFeAsO. Nat. Commun. 5:5738 doi: 10.1038/ncomms6738 (2014).